Immediate tool incorporation processes determine human motor planning with tools Human dexterity with tools is believed to stem from our ability to incorporate and use tools as parts of our body. However tool incorporation, evident as extensions in our body representation and peri-personal space, has been observed predominantly after extended tool exposures and does not explain our immediate motor behaviours when we change tools. Here we utilize two novel experiments to elucidate the presence of additional immediate tool incorporation effects that determine motor planning with tools. Interestingly, tools were observed to immediately induce a trial-by-trial, tool length dependent shortening of the perceived limb lengths, opposite to observations of elongations after extended tool use. Our results thus exhibit that tools induce a dual effect on our body representation; an immediate shortening that critically affects motor planning with a new tool, and the slow elongation, probably a consequence of skill related changes in sensory-motor mappings with the repeated use of the tool. Humans use a myriad of tools in their daily life ranging from a spoon to a golf club, without giving much thought. Contrary to the apparent ease, planning a movement with even a simple tool like a pointing stick is not trivial. To point to a board with a pointing stick, an individual’s brain has to first recognize the stick’s size, shape and dynamics, then locate its target in the visual and body coordinates, integrate this information with the stored body representation, before finally calculating the changes in limb angles required to make the movement to touch the target. It is generally accepted that, despite these complex and error-prone calculations, humans are dexterous with tools because of their ability to incorporate and use tools as extensions of their body [1] , [2] , [3] , [4] . However tool embodiment, evident as tool-induced lengthening of our perceived limb lengths, or body representation [5] , [6] , [7] , and extensions of the neural representation of the space around the body (so called peri-personal space) [2] , [3] , [8] , [9] , [10] , [11] , has been examined predominantly after extended use (~tens of minutes) of any tool. On the other hand, an individual can immediately switch from pointing on a board with the pointing stick to pointing with a much shorter pen without requiring any practice. This empirical fact suggests other immediate incorporation processes induced by tools. The existence of such immediate adaptations of body representations has been previously suggested [4] , but never proved. On the other hand, while studies have occasionally reported the peri-personal space to change even without specific tool training [2] , [12] , [13] , [14] , the effect of these changes on the subject’s motor behaviour with the tools have never been examined. Overall, whether and what immediate tool incorporation processes exist and if so, how they affect human motor behaviour is still not clear. In this study we aimed to isolate the immediate tool incorporation processes that determine motor planning with a tool. We first developed a two-choice forced discrimination task which allowed us to examine the immediate changes in the perceived free-arm reach space when an individual uses a tool. Next, using a novel tool-held reaching task, we examine the cause of the changes observed in the first task, and how these affect movement planning with tools. We used a haptic manipulandum in our tasks which enabled us to precisely measure the tool-held movements made by the subjects and equalize the dynamics across tools and no-tool conditions. Our results exhibit that tools induce immediate changes in our body representation; they immediately shorten our perceived arm length. The shortening is shown to critically determine the movement planning with the tool. Successful use of the tool with these initial planning processes are arguably key prerequisites for the long-term tool incorporation processes that have been regularly observed by previous studies [1] , [2] , [3] , [4] , [5] , [6] , [7] , [8] , [9] , [10] , [11] , [12] . Tools induce immediate perception changes In the first key-in-hole (KIH) experiment ( Fig. 1a ), subjects were required to make a short reaching movement holding a haptic manipulandum, followed by a reachability judgement task. The subjects received visual feedback of their hand position, tool and the target throughout a reach trial and were required to reach a target either with their hand cursor (no-tool trial) or with the tip of a virtual tool (the key) that was presented on a screen with its base over their right hand (in a tool trial). Immediately after every reach, the subjects were presented with the outline of their current key (the keyhole) at a random location on the table (see white key outline in Fig. 1a ). They were asked to judge if the keyhole was reachable with the key (and with the way they currently held the key) by pressing either a ‘yes’ or ‘no’ button with their free left hand. Note that the keyhole was distinct from the reach target. The subjects were required to hold their right hand at the reach target during the judgement task and after each judgement they went on to the next trial and never made an actual reach to the keyhole. Critically, the subjects were explicitly instructed that the keyholes always matched the size and angle of the held key. Therefore the judgement task in this experiment implicitly required the subjects to estimate if their hand could reach the base of the keyhole ( Fig. 1a ). The reachability judgement in the KIH task thus provided us with a way to estimate the immediate effects of the tool on the subject’s perception of his arm length, during tool (key) use. Note that the arm reaching in the KIH task only served as a contextual cue [9] , [15] for tool use and helped us magnify the tool incorporation effect [9] . 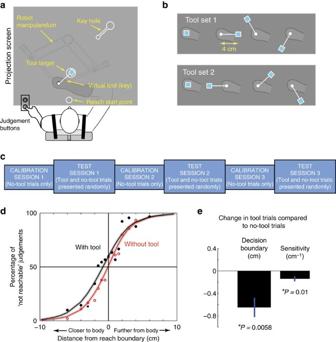Figure 1: KIH experiment. (a) The subjects held a manipulandum and were provided with virtual tools displayed on a screen over their hand. They were instructed to make a reaching movement with the tool from the reach start point to the tool target, following which they were presented with a ‘keyhole’. They judged if they can put their tool (key) into the keyhole using judgement buttons. (b) Each subject worked with one of two tool sets. (c) They performed three test sessions, each preceded by a calibration session. The calibration sessions included only ‘no-tool’ trials and was used to calibrate the reach boundary, about which the keyholes were presented in the following test session. (dande) The judgement from the tool and no-tool trials in the test sessions were assimilated over 10 subjects to create the psychometric curves and examine the immediate effect of tools on the reach space of one’s arm. We observed a significant change in both the decision boundary (T(9)=3.59,P=0.0058; two-tailedt-test on the individual differences between tool trials and no-tool trials) and sensitivity (T(9)=3.13,P=0.012; two-tailedt-test on the individual differences between the slopes of the tool and no-tool trials) between the tool and no-tool trials. Error bars represent s.e. Figure 1: KIH experiment. ( a ) The subjects held a manipulandum and were provided with virtual tools displayed on a screen over their hand. They were instructed to make a reaching movement with the tool from the reach start point to the tool target, following which they were presented with a ‘keyhole’. They judged if they can put their tool (key) into the keyhole using judgement buttons. ( b ) Each subject worked with one of two tool sets. ( c ) They performed three test sessions, each preceded by a calibration session. The calibration sessions included only ‘no-tool’ trials and was used to calibrate the reach boundary, about which the keyholes were presented in the following test session. ( d and e ) The judgement from the tool and no-tool trials in the test sessions were assimilated over 10 subjects to create the psychometric curves and examine the immediate effect of tools on the reach space of one’s arm. We observed a significant change in both the decision boundary ( T (9)=3.59, P =0.0058; two-tailed t -test on the individual differences between tool trials and no-tool trials) and sensitivity ( T (9)=3.13, P =0.012; two-tailed t -test on the individual differences between the slopes of the tool and no-tool trials) between the tool and no-tool trials. Error bars represent s.e. Full size image Each subject made 60 no-tool trials and 180 tool trials (divided equally between the three keys) over three sessions. To examine immediate effects of tool use on body perception, the tool and no-tool trials were mixed and presented randomly in each session, with three keys (tools of different orientation) presented randomly within the tool trials (see Fig. 1b , each subject received one of two tool set). The keyholes were presented between ±6 cm from the reach boundary (the origin of abscissa in Fig. 1d , also see Methods), which was calibrated before each session using a calibration session (experiment timeline shown in Fig. 1c ) where subjects made 45 (only) no-tool trials (details in the Methods section). The data from the judgement task in the randomly presented tool and no-tool trials were collected to generate a psychometric plot for each case. Figure 1d shows the psychometric plot of the keyhole reachability judgement averaged over the 10 subjects and the three test sessions. The data from the tool trials were combined as no differences were observed between the three keys in regards to the decision boundaries ( F (2,18)=1.36, P =0.28, repeated measures one-way analysis of variance (ANOVA)) or sensitivities ( F (2,18)=0.86, P =0.44, repeated measures one-way ANOVA) . The reachable space in the no-tool trials remained similar to the preceding calibration session (note that the red trace passes through the origin of the abscissa, two-tailed t -test, T (9)=0.218, P =0.83). However in the presence of a tool, the reachable space shown by the decision boundary of the hand shrunk across the tools ( T (9)=3.59, P =0.0058; two-tailed t -test on the individual differences between tool trials and no-tool trials, Fig. 1e ) such that the subjects judged closer keyholes to be not reachable. Furthermore, the sensitivity of the reach perception was also observed to decrease ( T (9)=3.13, P =0.012; two-tailed t -test on the individual differences between the slopes of the tool and no-tool trials, Fig. 1e ) in the presence of tools. As the tool and no-tool trials were mixed throughout the KIH experiment, the above observations clearly show that tools can immediately affect the subject’s perceived arm reach space without requiring any training with the tool; the perceived reach space decreased every time a subject held a tool and reverted back in the no-tool trials. Though interestingly, the immediate effect induced by the tools was seemingly contradictory to the perceived elongation of body representation [2] , [3] , [4] , [5] and peri-personal space [2] , [3] , [8] , [9] , [10] , [11] that has been observed by previous studies after the extended use of tools. Other than the fact that we looked for immediate tool effects, another difference of our study was in the characteristics of the tools used. While all the previous studies have consistently used tools that point away from the body (tending to extend the reach of the arm), our study also included tools that pointed towards the body when held in the hand (see tools in Fig. 1b ). To ensure that this qualitative difference in tool orientation was not the cause of the opposite observations, we conducted a subsidiary KIH (sKIH) experiment with eight subjects. The subjects in sKIH followed the same procedure as KIH subjects but, similar to previous studies, were only presented with tools that pointed away from the body (see Fig. 2a ). As we again observed no difference in the decision boundary ( F (2,14)=2.55, P =0.12, repeated measures one-way ANOVA) or sensitivity ( F (2,14)=0.08, P =0.93, repeated measures one-way ANOVA) across the tools, the data from the tool trials were combined for analysis ( Fig. 2b ). A significant and immediate reduction in the perceived reachable space was again observed in the sKIH experiment in the presence of tools ( T (7)=4.32, P =0.0035; two-tailed t -test on the individual differences between tool trials and no-tool trials, Fig. 2c ), though the sensitivity to reach perception was no longer observed to be different between the tool and no-tool trials ( T (7)=0.34, P =0.75; two-tailed t -test on the individual differences between the slopes of the tool and no-tool trials in Fig. 2c ). 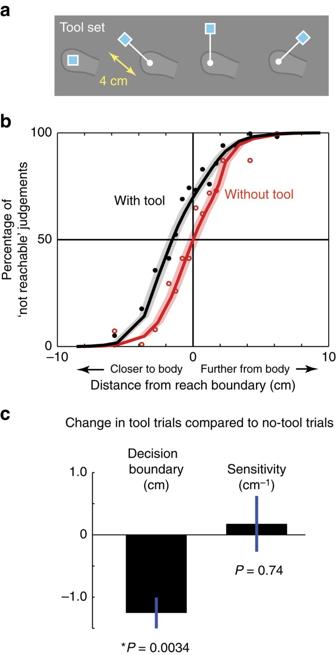Figure 2: sKIH experiment. Eight subjects participated in this experiment. The subsidary KIH experiment followed the same procedure and timeline as the KIH experiment. The only difference was in the tool set presented to the subject. (a) All tools presented in the sKIH pointed away from the body. (bandc) We observed a significant change in only the decision boundary between the tool and no-tool trials (T(7)=4.318,P=0.0035; two-tailedt-test on the individual differences between tool trials and no-tool trials). Error bars represent s.e. Figure 2: sKIH experiment. Eight subjects participated in this experiment. The subsidary KIH experiment followed the same procedure and timeline as the KIH experiment. The only difference was in the tool set presented to the subject. ( a ) All tools presented in the sKIH pointed away from the body. ( b and c ) We observed a significant change in only the decision boundary between the tool and no-tool trials ( T (7)=4.318, P =0.0035; two-tailed t -test on the individual differences between tool trials and no-tool trials). Error bars represent s.e. Full size image The use of virtual tools (like the one presented in the KIH and sKIH experiments) enabled us to equalize the dynamics across tools and no-tool conditions, as well as instantly switch between tool and no-tool conditions trial to trial. However, a critical concern remained regarding whether the observed reduction was a characteristic only while using virtual tools, and whether a similar reduction will also be observed with a real tool. To address this concern, we next conducted a third real-tool KIH experiment with 11 subjects, where we repeated the same KIH task but with subjects operating with a real tool in their hand ( Fig. 3a,b , and see Methods). We again observed a significant and immediate reduction in the perceived reachable space in the real-tool KIH experiment in the presence of tools ( T (10)=2.53, P =0.029; two-tailed t -test on the individual differences between tool trials and no-tool trials, Fig. 3 c,d ). Similar to the sKIH experiment, the no-tool decision boundary was again not different from zero ( T (10)=1.17, P =0.26). The sensitivity to reach perception was observed to be similar between the tool and no-tool trials ( T (10)=1.15, P =0.28; two-tailed t -test on the individual differences between the slopes of the tool and no-tool trials in Fig. 3d ; psychometric curves from each subject are shown in Supplementary Fig. 1 ). Quantitatively, the reduction with the 10-cm real tool was around 0.6 cm, which was considerably less than 1.1 cm observed with the 3-cm tools in the sKIH experiment. This difference was probably induced by the fact that the subject had to actively release their grip and switch between the ‘tool’ and ‘no-tool’ trials in the real-tool KIH, whereas these were changed immediately and without a grip change in the sKIH experiment (as the tools were virtual projections). Furthermore, the number of tool orientation was more in the sKIH experiment and may be a reason for the increased reduction in reach boundary observed in sKIH. 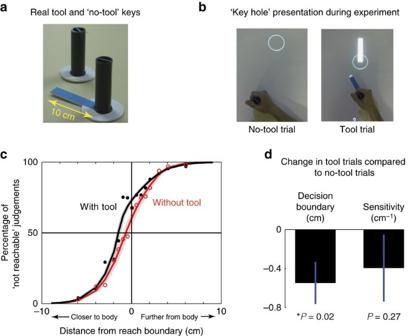Figure 3: Real-tool KIH experiment. The real-tool KIH experiment followed a similar procedure and timeline as the KIH experiment with 11 subjects manipulating real keys (tools). (a) The tool handle was made from plastic whereas the body was made with styrofoam. The ‘no-tool’ key consisted only of the handle. (b) The projected keyhole during a no-tool trial (left panel) and a tool trial (right panel). The subjects had to judge if the keyhole was reachable without making an actual movement to the keyhole. (candd) We observed a significant change in only the decision boundary (T(10)=2.53,P=0.029; two-tailedt-test on the individual differences between tool trials and no-tool trials) but not in the sensitivity (T(10)=1.148,P=0.28; two-tailedt-test on the individual differences between the slopes of the tool and no-tool trials) between the tool and no-tool trials. Error bars represent s.e. Figure 3: Real-tool KIH experiment. The real-tool KIH experiment followed a similar procedure and timeline as the KIH experiment with 11 subjects manipulating real keys (tools). ( a ) The tool handle was made from plastic whereas the body was made with styrofoam. The ‘no-tool’ key consisted only of the handle. ( b ) The projected keyhole during a no-tool trial (left panel) and a tool trial (right panel). The subjects had to judge if the keyhole was reachable without making an actual movement to the keyhole. ( c and d ) We observed a significant change in only the decision boundary ( T (10)=2.53, P =0.029; two-tailed t -test on the individual differences between tool trials and no-tool trials) but not in the sensitivity ( T (10)=1.148, P =0.28; two-tailed t -test on the individual differences between the slopes of the tool and no-tool trials) between the tool and no-tool trials. Error bars represent s.e. Full size image Parallel extension of perceived reach space Each test session in the KIH experiments was preceded by a calibration session ( Fig. 1c ) that was used to calibrate the no-tool reach space for that session. While the comparison between the tool and no-tool trials across test sessions helped us analyse the immediate perceptual changes in the presence of tools ( Figs 1 , 2 , 3 ), the comparison of the no-tool reach space perception across the three calibration sessions helped us analyse the long-term effects of tool use that exist in parallel to the immediate shortening of perceived reach space. We observed that the perceived free hand (no tool) reach boundary consistently increased across the calibration sessions of the KIH experiments ( Fig. 4 ). Although the increase did not reach significance in the KIH experiment (solid trace in Fig. 4 ; T (9)=2.08, P =0.076, two-tailed t -test of the individual difference between the first and last calibration sessions), the use of tools pointing away from the body led to a significant increase in the reach boundary across the calibration sessions in sKIH experiment (dashed trace in Fig. 4 ; T (7)=2.99, P =0.047 two-tailed t -test of the individual difference between the first and last calibration sessions) as well as the real-tool KIH experiment (thick dashed trace in Fig. 4 ; T (9)=3.01, P =0.015; two-tailed t -test of the individual difference between the first and last calibration sessions, one subject data was observed to be different by more than 2 × s.d. and was classified as a outlier). 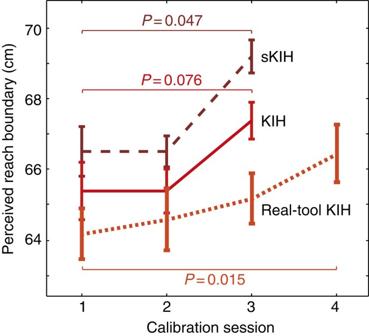Figure 4: Change of perceived reach boundary. The actual reach boundary calculated in the calibration sessions increased across the 10 subjects in KIH (solid red trace), 8 subjects in sKIH (dashed brown trace) and 11 subjects in real-tool KIH (dotted light orange trace) experiments. TheP-values represent the two-tailedt-tests performed on the difference in the percieved reach boundary in the first and the last calibration session across the subjects in each experiment. Error bars represent s.e. Figure 4: Change of perceived reach boundary. The actual reach boundary calculated in the calibration sessions increased across the 10 subjects in KIH (solid red trace), 8 subjects in sKIH (dashed brown trace) and 11 subjects in real-tool KIH (dotted light orange trace) experiments. The P -values represent the two-tailed t -tests performed on the difference in the percieved reach boundary in the first and the last calibration session across the subjects in each experiment. Error bars represent s.e. Full size image Tools effects and their cause Together the KIH, sKIH and real-tool KIH experiments concretely exhibit that tools induce a dual effect; an immediate reduction in the perceived reachable space when a tool is held, and a slow elongation of the reach space with the repeated use of tools, even when the tool trials were intermingled with no-tool trials. On the other hand, we believe that the change in sensitivity in the presence of tools arises from the interaction of the transients of the tool incorporation processes between the individual tool and no-tool trials. The transient interactions are more complex when the number of tools is more, leading to more noise in the perception (and loss of sensitivity). In agreement to this belief, we observe a decrease in sensitivity in the KIH task but not in the sKIH task where the tools are more similar (in terms of orientation) or in the real-tool KIH task where only one tool was used. As in this study we are interested in the change in body representation, we will concentrate on the reduction and its causes and leave the details regarding the sensitivity for future work. The KIH experiments required the subjects to view the keyhole and utilize their perceived arm length, or body representation, to estimate if the key was reachable. The reduction in the perceived reachability could thus have occurred due to either or both of two reasons; a change in body representation and specifically a reduction in the perceived arm length, or/and an elongation of the visually perceived keyhole distance probably due to the deformation of the peri-personal space [9] , [11] in the presence of tools. To concretely check the cause, we next investigated the effects of tools on the motor planning of arm movements made while holding the tool and compared it with the predictions made by models of changes in body representation and visual perception. Tool-held reach experiment In the second tool-held reaching (THR) experiment, we presented nine subjects with eight different tools, again as two different tool sets (see Fig. 5b ), and asked them to make movements to reach randomly presented targets (at a distance of 10 or 15 cm) with the tip of their tools. The targets were presented over one of six areas (see distribution of sample results from one subject superimposed in Fig. 5a in which each coloured dot represents the hand position with different tools). Unknown to the subjects, we offset the presented tool targets and equalized their hand movements such that correct movement with each tool required the subject to make the same hand movement as in the no-tool trial (see ‘Hand movement equalization’ section in Methods for details). Similar to the KIH experiments, the tool and no-tool trials were presented randomly across the THR experiment and at the start of each trial, a subject was presented with the visual feedback of the tool (and hand position), start position (of the hand) and the target for making the movement. However, in contrast to the KIH experiments, the visual feedback of the hand and tool in the THR experiment was switched off once the subject started to make a reach so as to avoid visual corrections during or after the movements. The target was visible to the subject throughout the trial. Therefore, the THR task required the subjects to plan their reach movement before each trial with the visible tool and target, and then make the movement relying solely on the motor planning (as no visual feedback was available during or after the reach). The THR experiment thus enabled us to observe the motor planning errors induced by the tools, which we then compared with error predictions made by models of body representation change (BRC model) and visual perception change (VPC model). 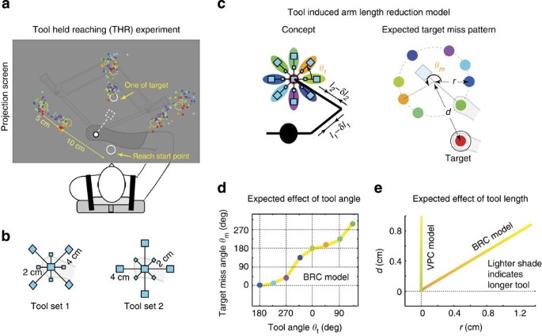Figure 5: THR experiment. (a) Experiment: Nine subjects performed reach movements to one of six hand targets holding a set of nine tools (eight tools and no-tool) presented randomly to them. The hand position data from a representative subject while holding different tools (colour code shown inc) is superimposed. (b) Each subject worked with one of two tool sets. The subjects were given visual feedback of their hand position, tool, start point and target before beginning each trial. The visual feedback of the tool and hand position were switched off once they started their movement. (c) Body representation change (BRC) model prediction: the BRC model assumes the tools lead to a proportional decrease in the perceived length of the upper arm and forearm. The colour code represents the tool orientation angles as shown in the left panel ofcsuch that for example, the hand positions after reach with tools of 0 degree (θt=0) are averaged and represented by light green, those with tools ofθt=45 are averaged and represented by orange and so on. The ‘no-tool’ condition is shown in red. The right panel ofcshows the predicted tool-held hand position with respect to the target (black circle) averaged over the same targets as in the experiment. The model predicted that no-tool trials to reach the target (see red disk in black circle). It predicted that the tools to lead to both an overshoot (d) of the target, as well as a deviation (r) along the length of the tool, such that (d) the target miss angleθmis roughly 180° flipped with respect to the tool angleθt. The example hand position without a tool and the hand and tool position for a tool ofθt=135 degrees is shown (not to scale). (e) The values ofranddwere predicted to increase linearly with the tool length (orange–yellow trace). On the other hand, the VPC model predicts a deformation in the visual perception leading to only a target offset proportional to the length of the tool (green–yellow trace ind). Figure 5: THR experiment. ( a ) Experiment: Nine subjects performed reach movements to one of six hand targets holding a set of nine tools (eight tools and no-tool) presented randomly to them. The hand position data from a representative subject while holding different tools (colour code shown in c ) is superimposed. ( b ) Each subject worked with one of two tool sets. The subjects were given visual feedback of their hand position, tool, start point and target before beginning each trial. The visual feedback of the tool and hand position were switched off once they started their movement. ( c ) Body representation change (BRC) model prediction: the BRC model assumes the tools lead to a proportional decrease in the perceived length of the upper arm and forearm. The colour code represents the tool orientation angles as shown in the left panel of c such that for example, the hand positions after reach with tools of 0 degree ( θ t =0) are averaged and represented by light green, those with tools of θ t =45 are averaged and represented by orange and so on. The ‘no-tool’ condition is shown in red. The right panel of c shows the predicted tool-held hand position with respect to the target (black circle) averaged over the same targets as in the experiment. The model predicted that no-tool trials to reach the target (see red disk in black circle). It predicted that the tools to lead to both an overshoot ( d ) of the target, as well as a deviation ( r ) along the length of the tool, such that ( d ) the target miss angle θ m is roughly 180° flipped with respect to the tool angle θ t . The example hand position without a tool and the hand and tool position for a tool of θ t =135 degrees is shown (not to scale). ( e ) The values of r and d were predicted to increase linearly with the tool length (orange–yellow trace). On the other hand, the VPC model predicts a deformation in the visual perception leading to only a target offset proportional to the length of the tool (green–yellow trace in d ). Full size image Tool-induced body representation change model In our KIH tasks we had observed that the decrease in perceived reachable space occurred irrespective of the tool orientation. Therefore in our body representation change (BRC) model, we assumed that only the tool length causes the changes in body representation. Specifically, the BRC model assumes that tool use leads to a reduction in the perceived arm length (upper arm l 1 →( l 1 − δl 1 ); forearm l 2 →( l 2 − δl 2 )) proportional to the length of the tool (concept shown in Fig. 5c , left panel). The model thus predicts that in the presence of a tool, the shoulder and elbow angles required for the reach movement will be planned with a reduced arm length and consequently, when these angles are executed with the actual arm, the model predicted the tool tips to miss the target in our experiment in a systematic pattern (see cartoon in the right panel of Fig. 5c , details of the simulation in methods). The BRC model predicted the tool tip and hence the hand position to not only overshoot the no-tool target along the direction of movement ( d in Fig. 5c ) but also deviate systematically along the length of the tool ( r in Fig. 5c ) such that, interestingly, the tool angles (represented by various colours in Fig. 5 ) are considered relatively well (see the miss pattern cartoon in Fig. 5c ). The predicted miss angles are presented in Fig. 5d . Furthermore, the model predicted both these errors ( r and d ) to increase linearly with the length of the tool (orange–yellow trace, Fig. 5e ). Tool-induced visual perception change model Next to model VPC, we again considered only the length of the tool so as to keep consistent with the BRC model. The VPC model assumes that holding a tool deforms the visual perception of an individual such that the visually observed targets are perceived farther away in proportion to the length of the tool. Though quantitatively opposite, this model is motivated by the reported decrease in perceived visual distance after extended use of tools [9] . The VPC model expects the targets in our task to be misperceived to be farther away in the presence of tools. Therefore, it predicts the subsequent movements with the tool (without visual feedback) to only overshoot the target ( d ) but show no deviation ( r ). The VPC model may thus be represented by y axis in Fig. 5e . As the model assumes the effect to depend on the length of the tool, it predicts the overshoot to increase with tool length (green–yellow trace in Fig. 5e ). Data and models The subject hand positions at the end of the reach through the THR experiment are analysed in Fig. 6 . First, across the subjects we observed that the no-tool trials reached every target ( T (8)<0.55, P >0.60, two-tailed t -tests on the ordinate and abscissa errors for each target over the subjects) with no consistent error relative to the target position. Therefore, for rest of the analysis, the hand positions for each subject were calculated relative to their mean no-tool endpoint. The inset of Fig. 6a shows the plot of the data from all our subjects across all the tools and targets during the THR experiment (see Supplementary Fig. 2 for separate plots for each target) plotted relative to their mean no-tool reach trials (red data point located at the origin). The colours represent the tool angles (colour coding same as in Fig. 5c ). In Fig. 6a inset and Supplementary Fig. 2 , we again notice the immediate effects of tool use on the arm movements—even though the tool and no-tool trials were mixed, the tool trials show a systematic error depending on the tool orientation (shades of blue, green, purple and orange) with respect to the no-tool trials (red data). The subjects consistently overshot the targets and also deviated along the length of the tool. These errors correspond well to the BRC model, which predicted the target miss angle θ m to be roughly 180° flipped with respect to the tool angle θ t ( Fig. 6a ), although a small but significant difference of the miss angle from the model prediction were observed for three out of eight tool angles (two-tailed t -tests, T (8)>2.35, P <0.05 for θ m =45, 90, 270). The overshoot ( Fig. 6b ) was also well explained by the BRC model for the three cases of no tool, a 2-cm tool (the ratio of d/r was not different from the model prediction; two-tailed t -test gave T (8)=0.05, P =0.96, Fig. 6b ) and 4-cm tool ( T (8)=0.34, P =0.70). On the other hand, the miss behaviours were significantly different from the VPC model ( T (8)=7.03, P =10 −4 , two-tailed t -test for 2-cm tools, and T (8)=4.44, P =0.002 for 4-cm tools, relative to the y axis). 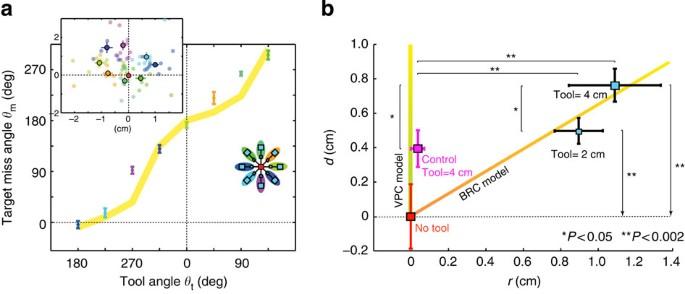Figure 6:THR experimental models and data. The model predictions have been replotted with the experiment data superimposed on top. (a) The inset shows the individual subject data averaged over the targets with the colour code representing the tool angle and the large circles representing the across subject average. The data is plotted relative to the mean no-tool reach positon (red plot on inset origin). The target miss angle of the collected data (from the inset) is plotted (different colours correponding to the colour code) over the BRC model prediction of the miss angles (yellow trace ina). The experiment data matched the model well, though there was a small but significant difference for three tool orientations (two-tailedt-tests,T(8)>2.35,P<0.05 forθm=45, 90, 270). (b) The ratio of the overshoot (d) is plotted against the deviation (r) from the experiment matched with the BRC model (orange–yellow trace) for both the 2-cm tools and 4-cm tools (two-tailedt-test gaveT(8)=0.05,P=0.96) and 4-cm tool (T(8)=0.34,P=0.70). On the other hand, the miss behaviours were significantly different from the VPC model (green–yellow) both for the 2-cm tool (T(8)=7.03,P=10−4, two-tailedt-test relative to theyaxis) and 4-cm tool (T(8)=4.44,P=0.002, two-tailedt-test relative to theyaxis). The data from the control THR experiment is plotted in pink. Radial deviation was absent in the control task (two-tailedt-test for the difference ofrvalues from zero;T(9)=1.17,P=0.27). A target overshoot was observed (T(9)=3.71,P=0.0048, two-tailedt-test) in the control but it was less than the THR experiment for the same tool length (two-sample two-tailedt-test between thervalues from Control and THR experiments;T(17)=2.66,P<0.017). Error bars represent s.e. Figure 6: THR experimental models and data . The model predictions have been replotted with the experiment data superimposed on top. ( a ) The inset shows the individual subject data averaged over the targets with the colour code representing the tool angle and the large circles representing the across subject average. The data is plotted relative to the mean no-tool reach positon (red plot on inset origin). The target miss angle of the collected data (from the inset) is plotted (different colours correponding to the colour code) over the BRC model prediction of the miss angles (yellow trace in a ). The experiment data matched the model well, though there was a small but significant difference for three tool orientations (two-tailed t -tests, T (8)>2.35, P <0.05 for θ m =45, 90, 270). ( b ) The ratio of the overshoot ( d ) is plotted against the deviation ( r ) from the experiment matched with the BRC model (orange–yellow trace) for both the 2-cm tools and 4-cm tools (two-tailed t -test gave T (8)=0.05, P =0.96) and 4-cm tool ( T (8)=0.34, P =0.70). On the other hand, the miss behaviours were significantly different from the VPC model (green–yellow) both for the 2-cm tool ( T (8)=7.03, P =10 −4 , two-tailed t -test relative to the y axis) and 4-cm tool ( T (8)=4.44, P =0.002, two-tailed t -test relative to the y axis). The data from the control THR experiment is plotted in pink. Radial deviation was absent in the control task (two-tailed t -test for the difference of r values from zero; T (9)=1.17, P =0.27). A target overshoot was observed ( T (9)=3.71, P =0.0048, two-tailed t -test) in the control but it was less than the THR experiment for the same tool length (two-sample two-tailed t -test between the r values from Control and THR experiments; T (17)=2.66, P <0.017). Error bars represent s.e. Full size image Control for misperception of tool length Next we conducted an important control experiment to show that the deviations ( r ) observed in our task were not due to a visual misperception of the tool length by the subject. A separate group of 10 subjects participated in the control experiment. While in the THR task the subjects had no feedback of either their hand position or the tool during the reach, the subjects in the control experiment were provided the visual feedback of only their hand position (and not the tool) during the reaching movement. It was observed that in the presence of the visual feedback of their hand position, the subjects could consistently reach the target with the tool (see pink plot in Fig. 6b ). The radial deviation r was absent (two-tailed t -test for the difference of r values from zero; T (9)=1.17, P =0.27). Though a target overshoot was still observed ( T (9)=3.71, P =0.0048, two-tailed t -test), it was significantly less than in the THR experiment for the same tool length (two-sample two-tailed t -test between the r values from Control and THR experiments; T (17)=2.66, P <0.017). Critically, the absence of deviations in the presence of visual feedback of the subject hand in this control experiment clearly exhibits that the deviation observed in the THR were not due to a visual misperception of the tool length but due to the misperception of the hand (body) position. Previous studies investigating tool embodiment in primates have repeatedly shown changes in the peri-personal space and body representation induced by repeated use of a tool. However, these effects induced by protracted tool use do not explain our ability to immediately use a tool that we have just picked up. In this study we exhibited that tool incorporation includes immediate perception changes that are arguably critical to this ability. We started with a simple two-choice discrimination task (KIH experiment) similar to the study of Bourgeois et al . [16] and exhibited that tools can induce an immediate change in the perceived reachable space of the tool-free arm. Next, using a movement task in the THR experiment, we exhibited that the changes observed by us are well explained by changes in body representation in the presence of a tool. Critically, in both experiments we utilized tools of different size and orientation and mixed the tool and no-tool trials. This ensured that the changes we observed were immediate effects associated with tool use and different from the changes in body representation due to repeated use of a same tool. However interestingly, the effects observed in our experiment were opposite to that observed by previous studies; we observed that the perceived arm length shortens immediately in the presence of a tool, whereas previous studies have exhibited that the repeated use of a tool elongates the body representations [5] , [6] , [7] and peri-personal space [2] , [3] , [8] , [9] , [10] , [11] . We hypothesized the differences between our observations and that of the previous studies to be due to the presence of two parallel processes of different time constants during tool use; a fast shortening process in the presence of a tool and a slow elongation process resulting from the extended use of tools. This hypothesis is supported by our observations that, in addition to the immediate shortening ( Figs 1d , 2b and 3c ), tool use also results in a slow increase in the perceived reach boundary across the KIH calibration sessions ( Fig. 4 )—a result that agrees with the previous reported extensions of body representation. So what can be the reason for the presence of two parallel tool-induced adaptations of the body representation? When a tool is used repeatedly, the association between the control commands to the arm while holding the tool and the sensory signals received with the tools can lead our central nervous system to develop new sensory–motor associations; a process which was arguable the cause of the extensions in body representations observed by previous studies. This long-term association probably helps reduce the computational time and cost of motor planning with the tools and determines our skill with the tool. On the other hand, this incorporation by association is expected to take at least few trials and not be very useful for the immediate use of a new tool after a tool change. Using a new tool, like for reaching in our THR task, requires an immediate estimation of the tool kinematics followed by movement planning corresponding to the kinematics, and finally the movement execution aided by the visual feedback. Especially the visual feedback, which is most active at the end of the reach [17] , is probably the key factor that determines successful reach with a new tool. For efficient visual feedback, the one crucial requirement is that the hand (and tool) movement does not occlude the view of the reach target. Considering the fact that the tool-held reaching can be affected by the visual perception errors, motor planning noise [18] and motor execution noise [19] , an obvious efficient strategy would be to plan the movement away (deviate) from the target ( r in Fig. 5c ), make sure the target is not occluded and then rely on the visual feedback to bring the tool to the target at the end of the reach. We suggest the shortening of limb representation to be a deliberate procedure adopted by the human central nervous system to achieve an approximate deviation ( r in Fig. 5c ); where the deviation is calculated by utilizing the estimate of one’s own motor noise [20] but without requiring accurate visual calculations of the tool characteristics (especially the orientation). In fact in partial support to the deliberate nature of the arm shortening we find a significant correlation ( R =0.37, P <0.01, Supplementary Fig. 3 ) between an individual’s motor noise, measured in the no-tool trials, and the associated deviation ( r ) in the tool trials in our THR experiment. To our knowledge, this observation provides the first direct evidence to show that tool-induced changes in body representation have a functional role in motor control with the tool. While the observations in this study are well explained by the perceived shortening of the limb lengths (BRC model) and not by a simple deformation of visual perception (VPC model), the results may be explained if we take a more complicated VPC model considering simultaneous elongation (along the movement) and warping (along the tool length) of visual perception in the presence of tools [11] . However, two aspects of our results suggest the changes in body representation as the major source of movement errors with tools. First, the elegant explanation of the seemingly complex target miss patterns provided by a simple body representation change model ( Fig. 6 ); And second, the dependence of the deviation on an individual’s internal motor noise parameters ( Supplementary Fig. 3 , as discussed in the previous paragraph). However having said that, we cannot conclude that the changes in body representation were the sole cause of the effects observed in our experiments. In fact, the continued presence of target overshoots in the control experiment (pink plot of Fig. 6b ), model errors in specific tool orientations ( Fig. 6a ) and a requirement of a scaling factor in our BRC model (see Methods) exhibit that, either the BRC model can be optimized by considering additional transformations in its tool estimates and/or additional tool-induced processes, probably related to changes in the visual perception and peri-personal space, are also active during tool use. Critically, whatever the relative quantitative contribution of the causes, the THR experiment clearly exhibits the presence of the immediate tool incorporation process and that it effects tool-held movements, which is the main goal of this study. Though the complete definition of a ‘tool’ is still not clear and the classical definition by Beck [21] is considered too strict [22] , it is generally believed that tools cause a physical effect on the environment, and a consequent haptic feedback to the user. To this effect, tool-induced perceptual effects have been observed to be different in the presence and absence of physical interactions; when a tool is used to estimate the size of an object rather than lift it [23] and when a stick rather than a light pointer is used to point to a line centre in a line bisection task [2] . Interestingly in our tool tasks, which may be considered similar to pointing, we observed tool incorporation effects even in the absence of a specific physical effect on the environment. However, though the tool use in our tasks did not lead to a physical consequence, they resulted in changes in the experiment environment; Tool reach resulted in the appearance of the keyhole in the KIH tasks, and tool reach was followed by the subject hand being brought back to the start position by the robot manipulandum in the THR task. We believe that these changes were perceived by the subjects as effects being caused by their tool use, and this causal perception was responsible for the tool incorporation observed in our tasks. Therefore our results support the definition suggested by Holmes et al . [22] and suggest that the sensory perception of an effect (even non-haptic) as being caused by an object held task is key for the object to be perceived as a tool. Incorporation of tools into one’s body has been the general terminology regularly used for perceived extensions in one’s body and environment representations in the presence of tools, and considered to be critical in one’s ability to use tools [1] , [3] , [4] . Our results indicate that the incorporation of tools is a more complex process than previously known and includes multiple processes of different time scales. Understanding the human ability of tool use requires not only the isolation of these perceptual processes but also understanding their interactions with the movement control in the presence of the tools [24] . The immediate processes induced by the tools, like the one exhibited in this study, are of critical importance in this regard because they determine the successful use of a new tool. It is only in the presence of these initial successes that the sensory–motor associations in the presence of the tool can be reinforced [25] and lead to long-term ‘incorporation of the tool into one’s body’. Subjects Forty-nine subjects, aged 23–42 years, participated in our five experiments. The subject numbers were kept to around 10 per experiment corresponding to previous studies on arm-reaching and tool-induced perception changes. All participants were right-handed as assessed by the Edinburgh Handedness Inventory (Oldfield, 1971). The subjects gave informed consent for their participation in the experiments, which were conducted according to the principles in the Declaration of Helsinki and approved by the ethics committee at the National Institute of Information and Communications Technology. In all our experiments, subjects were seated comfortably on a chair and strapped to the position using seat belts (See Fig. 1a ). They held the handle of TVINS robot manipulandum with their right hand and were provided with the visual feedback of their hand position (cursor) and targets on a projection screen that covered their hand ( Fig. 1a ). In the tool trials, a virtual tool of particular orientation and size was projected at the hand position. KIH experiment Ten subjects participated in this experiment. The KIH experiment consisted of nine sessions starting with three training sessions to acclimatize them to the manipulandum and experiment, followed by three sets of alternating calibration and KIH sessions (data from these KIH sessions are presented in Fig. 1 ) The subjects first started with a session where they were asked to make 50 reaching movements holding the manipulandum to visual targets presented randomly on the screen and at a distance of 10 cm from the start point. The subjects were provided with a ‘go’ signal to make the movement but were specifically told there was no particular movement speed required and that they could move their hands at any chosen comfortable speed. This session helped the subjects get used to making movements holding the manipulandum. In the next training session, the subjects were provided with different tools and asked to make reaching movements to reach targets with the tip of their tool. They made a total of 25 movements with four different tools and without a tool. The tools presented in this session were different from those presented in the experiment after. Finally in the third training session, the subjects first made a reaching movement either with and without the tool (which we called a key) to a reach target. After the reach, their hand was held at the reach target by the robot and they were presented with an outline of their tool (or keyhole) on the projection screen and asked to judge, without making an actual movement, if their hand and key could reach the presented keyhole. They made their judgement by pressing on one of the ‘yes’ or ‘no’ buttons with their index finger of their left hand ( Fig. 1a ). Critically, the subjects were explicitly instructed that the keyholes always matched the size and angle of the held key. Therefore the judgement task in this experiment implicitly required the subjects to estimate if their hand could reach the base of the keyhole ( Fig. 1a ). The KIH task thus provided us with a way to estimate the changes in the body representation when holding a tool (the key). The subjects performed 25 trials in this training session. The calibration sessions were used to calibrate the ‘reach boundary’ for a subject. The calibration session consisted of two sub-sessions. In the first sub-session, the subjects made 15 reach movements without tools (all no-tool trials) to a target presented 20 cm away and with full visual feedback. This section was added to enable the subjects to ‘stretch their arm’ after complaints by subjects during our pretests (used for designing the experiment) that they felt constrained as they never got to stretch their arm for about an hour. In the second sub-session, the subjects made 45 movements without a tool (all no-tool trials) to reach targets presented randomly at 10 cm from the start position, following which they were presented with reach circles similar to the cursor and asked to judge if it was reachable or not. The reach circles were presented pseudo randomly between 52 and 80 cm from the shoulder (a range in which we found the subject arm lengths to lie in). The psychometric curve plotted with this data was used to define the reach boundary ( B c centimeters) as perceived by each subject before each KIH session. Finally in the KIH session ( Fig. 1 ) subjects were asked to make a short arm-reaching movement (of 10 cm) to touch a target either with their hand cursor (no-tool trial) or with the tip of a virtual tool (the key) held in their right hand (tool trial). The tool and no-tool trials were mixed and were presented randomly. In addition, three keys were presented randomly within the tool trials (see Fig. 1b , each subject received one of two tool set). Similar to the calibration session, after the reach, the subjects were asked to hold their hand position at the reach target (the robot held their arm as well) and then presented with the keyhole at a random location on the table (see white key outline in Fig. 1a ). They were asked to judge if the keyhole was reachable with the key (and with the way they currently held the key) by pressing either the ‘yes’ or ‘no’ button with their free left hand. The keyholes were presented at one of 15 locations over a range of −6 to +6 cm around the calibrated reach boundary ( B c ) at distances of { B c +[−6, −4, −3, −2, −1.5, −1, −0.5, 0, 0.5, 1, 1.5, 2, 3 ,4 ,6]} cm. The calibration and KIH sessions were repeated three times. We were thus able to analyse both the change in reach boundary across the three calibration sessions ( Fig. 4 ) and the change in the reach boundary within the KIH sessions between the tool and no-tool trials ( Fig. 1d ). Subsidiary KIH experiment Eight subjects participated in the sKIH experiment. The sKIH experiment followed the exact same procedure as the KIH experiment with the only difference being in the key orientation. All tools (keys) presented to the subjects in sKIH experiment pointed away from the body (see Fig. 2 ). Real-tool KIH experiment To check that the results we observe are not specific to the use of virtual tools, we also performed the KIH task with a real tool. 11 subjects participated in this experiment. Two tools (keys) were used in this real-tool KIH task. The ‘tool’ key was constructed by using a plastic handle with a round base and styrofoam tool head of 10 cm length. The ‘no-tool’ key was identical except that it did not have a tool head (see Fig. 3a ). The plastic and styrofoam ensured that the tools were very light and could smoothly slide over our experiment table. The weights of the two keys were equalized. The subjects worked on the same table (robot-visual feedback setup) as the other KIH experiments, but instead of holding a robot under the table with a virtual tool projection, they used a real tool that they could move by sliding on the table ( Fig. 3a,b ). The subjects followed the same experimental procedure as the KIH task, with a few changes. The subjects were asked to grip the tool such that the tool axis was aligned with their forearm. As the tool was 10 cm long, the reach targets were presented further at 20 cm for the tool conditions and at 10 cm for the no-tool condition to roughly equalize the arm movements to the previous KIH tasks. Before the start of each movement, they were instructed to pick up and use one of two keys ( Fig. 3a ) according to the presented shape of the start position. A circular start point indicated that they have to use the ‘no-tool’ key to make the reach, whereas an elongated starting location (same length as the real tool key) indicated that they had to pick up the tool key and align it to the start before making a reach. As we no longer use the manipulandum and were unable to judge when the reach is completed, the key presentation was fixed at 0.85 s after the start of the reach. This delay was found to be long enough for the subjects to make a reach at a comfortable speed and similar to the reaches in the previous KIH tasks. The axis of the keyhole was always presented aligned along a line joining the shoulder and keyhole location. The other instructions and procedure regarding the reach to a given target and the subsequent reachability judgement remained same as before. Tool-held reach experiment Ten subjects participated in the THR experiment. One subject was omitted as he felt sleepy and missed majority of his trials in a session. None of the subjects had experience in either of the KIH experiments. The subjects started with a training session in which they made 48 movements without a tool. This session enabled subjects to acclimatize themselves to make reaching movements with our manipulandum. The subjects were provided with the visual feedback of the target, hand position and tool at the start of the reach movement but the visual feedback of the hand position and tool were switched off as soon as the hand left the start position. Therefore, the subjects could not rely on the visual feedback to reach the target but had to rely on their movement planning performed before the reach, to make each reach. They were asked to make a `one-shot' reach movement and maintain their hand at the reached position until the manipulandum brought their hand back to the start position. The point where their velocity fell below 0.02 ms −1 was considered as the movement end. This threshold was determined by previous motor reach experiments in the lab. The visual feedback of the hand and that of the new tool were switched on again when the subject returned back to the start position for the next trial. After the training session, the subjects participated in four sessions, in which they made 108 movements each, with similar visual feedback conditions as they had trained for. In each trial, a subject was presented with one of eight tools (from one of two tool sets, see Fig. 5b ), to reach one of the targets with the tip of the provided tool. In total, each subject made 432 movements over the four sessions either without a tool or with one of eight tools (48 trials of each). We used two tool sets, with five subjects working with each. In addition, 30 no-tool visual trials (where the vision of the hand was kept on through the movement) were included randomly across the four sessions to ensure that there is no slow drift in the target reaches. These trials were not considered in the data analysis. Hand movement equalization Note that to ensure that the change in intended hand movement with each tool (to the same target) does not influence the results, we equalized the required hand movements made with each tool to the same hand target as follows. We decided the hand targets (see white dashed circle in Supplementary Fig. 4 ) first and offset the presented tool target corresponding to each tool (white solid circle in Supplementary Fig. 4 ) such that the hand movement with each tool becomes same ( Supplementary Fig. 4 shows the tool target presented with each tool. Note that they all lead to the same hand movement if performed correctly). The subjects were unaware of this modification and did not realize that their hand movements were same while reaching with a different tool towards the same direction. Control tool-held reach experiment To check that the subjects do not visually misperceive the length of the tool, we performed a control THR experiment with 10 subjects. The subjects in the control performed the same THR task, but were provided with the visual feedback of the hand cursor (but not of the tool) when they made the reaching movement. The logic behind this experiment was that if the subject visually misperceived the length of the tool, then the errors we observed in the THR experiment would remain in the control. On the other hand, if they misperceived their hand position in the THR experiment, then behaviour in the control would be different from the THR experiment. Body representation change model The BRC model assumes that holding a tool leads to one’s arm (upper and forearm) being perceived shorter than usual. Note that as we lock the wrist position, in the following explanation we assume the wrist to be an extended part of the forearm. Given the start angles, the model assumes that the plan for the movement with the tool is developed with a (misperceived) shortened upper and forearm. It predicts that when the joint angles calculated with this plan is applied with the real arm, it would lead to target misses. The model assumed the upper arm and forearm shorten in the presence of a tool as follows: Where represent the perceived upper arm and forearm lengths in the presence of the tool, while the represent the normal/real perception of the upper arm and forearm lengths when no tool is present. l t represents the tool length while ρ (=0.013) represents the linear factor that determines how the tool affects the perceived limb lengths. We took l ua =30 cm and l fa (forearm+closed wrist)=35 cm. At the start of a reach trial, a subject is shown his hand position, tool and the target. Given the reach target as ( X tar , Y tar ), start position of hand as ( X st , Y st ) and assuming the visual tool length ( l t ) and tool angle ( θ t ) was judged perfectly, the subject can calculate the tool tip coordinates as Our task was planar, where the subjects could use only their shoulder (shol) and elbow joints. The fixation of the hand on the manipulandum prevented them from using their wrist. Therefore we can uniquely calculate the joint angle required to perform the reach. The BRC model assumes that the subject estimates the target reach and tool length in terms of a change in their joint angles, and calculates the required hand movement to make the reach by subtracting the joint angle corresponding to the tool length from the required joint angles to reach the tool target with the hand (without the tool). The model assumes that the subject calculates the tool length before the movement start in terms of their joint angles (because this is the only time the tool is visible) as: where and Invkin( X , Y , l ua , l fa ) represents the inverse kinematics function given by: with the appropriate coordinate considerations. Note that the start position is available to the subject through both his proprioception and inverse kinematics of visual hand position and although his actual perception is probably a combination of the two, here we assume that vision dominates this estimation process [26] . The joint angles required to reach an observed tool target with the hand (without the tool) are given by The overall joint angle changes required to reach the target (holding the tool) with the tool tip are estimated by: k shol and k elbow are scaling factors used to fit our data quantitatively. Finally, the movement expected due to the misplan (with the misperceived upper arm and forearm lengths) can be calculated as Note that we use the real limb lengths in this calculation. forwkin( θ shol , θ elbow , l ua , l fa ) represents the forward kinematics function given by: The concept of the BRC model is shown in the left panel of Fig. 5c , and its average predictions over the same tool targets as in our experiment are shown in Fig. 5d,e . The model uses three parameters. ρ adjusts the effect of the tool on the arm length and was set to 0.013. k shol and k elbow were used as scaling factors for the shoulder and elbow angle changes. k shol =1 (no scaling) and k elbow =1.3 gave optimal fit on the averaged data. We note here that even though the scaling factors can be used to explain some deviations even in the absence of any tool-induced effects, the experiment data is matched, especially in terms of the overshoot, only in the presence of a tool-induced reduction in limb perception (that is, ρ >0). Although it is not completely clear why a scaling occurs in our task, we believe it can come from the online control during the task. While we perform the joint angle identification only at the start of the movement, a similar process is probably repeated by a subject through his movement, leading to accumulation of the error. This would explain why the scaling is present only in the tool trials and does not affect the no-tool trials. It is also interesting to note that the scaling is required more on the elbow angles even though over the targets both the shoulder and elbow contribute in making the reach. This indicates to probably a differential effect on the lower and upper arm due to the tool, similar to the report by a previous study [5] . Visual perception change model The VPC model was assumed as a linear extension of the perceived target distance along the direction of movement. The change in perceived reach target position is assumed to be additive and proportional to the length of the tool: where (X tar , Y tar ) represents the actual target coordinates, while (X tar VPC , Y tar VPC ) represents the perceived target coordinates. l t represents the tool length and ϕ represents the movement angle (angle of the line joining the start position to the target with respect to the x axis). β is a constant that was calculated as 0.175 from the data of the KIH experiment (change in decision boundary/tool length ⩾ 0.7/4=0.175). Model constraints Critically, it should be noted that here we have examined (in both BRC and VPC) minimal models with minimal parameters. These minimal models were sufficient for us to distinguish whether changes in limb perception or changes of visual perception were causes of the observations in our study. However while the minimal BRC model, where the parameters were tuned on the averaged data, can qualitatively explain target overshoot and deviation across the workspace ( Supplementary Fig. 2 ), and the average subject behaviour ( Fig. 6 ), it does not capture local quantitative variations in the subject behaviour. For example, the model predictions exhibit higher errors in certain tool angles ( Fig. 6a ) and certain targets (right targets of Supplementary Fig. 2 ). Therefore the BRC model does not represent the complete model of human tool use. As mentioned in the discussion, the model requires to consider additional tool related effects including possible interactions between tool orientation and movement direction to explain the complete human tool behaviour across the entire tool-arm workspace. Analysis of KIH data The reachability judgement data from a tool and no-tool trials were collected together and averaged for each subject in 15 bins according to the distance from the reachable boundary. For each subject, the averaged judgement over the 15 bins was fitted with an exponential curve of the form Where J represents the percentage not reachable judgement, 0 representing ‘reachable’ and 100 representing ‘not reachable’, parameter a represents sensitivity and b the decision boundary. δ represents the distance from the reach boundary where the keyhole was presented. The decision boundary calculated in each calibration session without the tool was used as the reach boundary in the subsequent KIH session. The decision boundary (perceived reachable space) from the calibration sessions are plotted in Fig. 4 . The difference between the decision boundaries in the tool and no-tool trials within the KIH sessions were collected across the subjects and a t -test was used to determine the significance of the change. The subject averaged psychometric curve was plotted at the solid trace in Figs. 1d , 2b and 3c . The shaded region represents the ±s.e. of the decision boundary. Analysis of the THR data For each subject, the hand position of the no-tool reach trials was averaged for each target. Across the subjects and targets, the no-tool reached the target ( T (9)<0.55, P >0.60, two-tailed t -test on the ordinate and abscissa errors for each target over the subjects) with no consistent error with relative to the target position. The rest of the analysis for each subject was thus done relative to the mean no-tool endpoint. For each subject the hand position of the reach made with each tool of the eight tools was considered relative to the mean no-tool reach endpoint and averaged across the six targets. The averaged data from each subject and tool orientation for each target is presented in Supplementary Fig. 2 . The data averages over the targets was plotted in the inset of Fig. 6a and coloured according to the tool angle with the colour code shown in Fig. 5c . For calculating the target overshoot ( d ) and deviation ( r ), the endpoints hand positions averaged across the six targets was plotted individually for each tool length and for every tool angle as in the inset of Fig. 6a . The average of the ordinate and abscissa over the different tools was considered as the ‘centre’ where the subject tended to reach with a tool. The angle of the line joining the center and each of the tool reach points was averaged across the six targets for each subject. The subject average for each tool was plotted in Fig. 6a . The distance of the centre from the no-tool reach endpoint gave the target overshoot ( d ) for that subject. The average distance of the hand reach position with each tool from the centre was used as the deviation ( r ) for the subject. The average d and r across the subjects was plotted in Fig. 6b . A similar procedure was followed to plot the data from the THR control experiment in Fig. 6b . How to cite this article: Ganesh, G. et al . Immediate tool incorporation processes determine human motor planning with tools. Nat. Commun. 5:4524 doi: 10.1038/ncomms5524 (2014).